Visible-frequency asymmetric transmission devices incorporating a hyperbolic metamaterial Asymmetric electromagnetic transmission has been recently demonstrated using Lorentz-reciprocal devices, which exploit a variety of patterned structures of linear materials to break spatial inversion symmetry. However, nanofabrication challenges have so far precluded the fabrication of passive transmission structures with highly asymmetric responses at visible frequencies. Here we show that high-contrast asymmetric transmission of visible light can be provided by a planar device of wavelength-scale thickness incorporating a pair of nonsymmetric subwavelength gratings and a passive hyperbolic metamaterial engineered to display a transmission window centred at a lateral spatial frequency substantially exceeding the diffraction limit. Fabricated devices designed for operation at central wavelengths of 532 and 633 nm, respectively, display broadband, efficient asymmetric optical transmission with contrast ratios exceeding 14 dB. Owing to its planar configuration, small footprint and passive operation, this reciprocal transmission approach holds promise for integration within compact optical systems operating at visible frequencies. Asymmetric transmission using reciprocal electromagnetic devices has recently become a thriving research topic owing to potential applications in integrated photonic systems for communications and information processing [1] , [2] , [3] , [4] , [5] , [6] , [7] , [8] , [9] , [10] , [11] , [12] , such as, directionally-sensitive beam splitting [2] , [3] , multiplexing [4] and optical interconnection [7] , [8] . This Lorentz-reciprocal effect is characterized by the high contrast between forward and reverse transmission under illumination from anti-parallel directions. Though reciprocal asymmetric transmission devices cannot be used for functions attainable only with non-reciprocal-active devices, such as optical isolation [13] , [14] , [15] , [16] , they have unique advantages such as small footprint, broad asymmetric transmission bandwidth and passive operation. Asymmetric transmission can be achieved through the use of artificial structures, such as, nonsymmetric gratings [2] , [3] , [4] , [5] , [6] , [11] , [12] , photonic crystals [7] , [8] and split-ring resonators [1] , [9] , [10] which break spatial inversion symmetry. Nevertheless, fabrication and alignment challenges associated with the intrinsic complexity of such approaches have not so far enabled structures with an efficient asymmetric transmission response at visible frequencies. Hyperbolic metamaterials—metallo-dielectric structures engineered on a deep-subwavelength scale to effectively act like a homogeneous electromagnetic medium with a highly anisotropic, hyperbolic spatial-frequency response—have become a topic of significant research interest in recent years [17] , [18] . These materials offer an efficient way to manipulate the propagation of light to yield a number of novel and exotic phenomena, such as, negative refraction [19] , [20] , [21] , [22] , [23] , super-resolution imaging [24] , [25] , [26] , enhanced optical absorption [27] , [28] and spontaneous emission [29] , [30] . In this work, we leverage a visible-frequency hyperbolic metamaterial to implement a planar device of wavelength-scale thickness able to enforce highly asymmetric, broadband transmission of transverse-magnetic (TM) polarized visible-frequency light under illumination at normal incidence. The proposed device consists of a sub-micrometre-thick slab of hyperbolic metamaterial decorated on each side (‘A’ and ‘B’, respectively, Fig. 1a ) with parallel metal diffraction gratings (‘grating A’ and ‘grating B’, respectively), each having a different subwavelength pitch. The spatial-frequency response of both metamaterial and gratings are designed such that light is transmitted from free-space on side A into free-space on side B, when the device is illuminated at normal incidence on side A, but blocked from transmission into free-space on side A, when the device is illuminated at normal incidence on side B. At a given frequency ( ω 0 , corresponding to free-space wavelength λ 0 and wavevector magnitude k 0 =2π/ λ 0 ), transmission through the metamaterial when illuminated on side A is mediated by a pair of oblique, laterally counter-propagating modes, with tangential spatial frequencies ± k x (oriented parallel to the metamaterial surface and normal to the grating pitch) that are substantially larger in magnitude than k 0 . These modes couple from normally incident light on side A to outgoing oblique light on side B through the action of gratings A and B. Conversely, normally incident light on side B is coupled to a pair of non-propagating, evanescent modes located within the tangential-wavevector bandgap of the hyperbolic metamaterial, which thus acts as a zero-order transmission barrier. 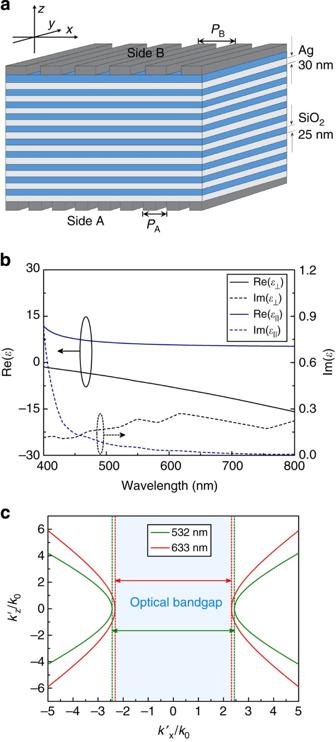Figure 1: Hyperbolic metamaterial composed of alternative Ag and SiO2thin layers. (a) Schematic diagram of the Ag/SiO2metamaterial devices. (b) EMT-derived effective permittivity⊥and||for metamaterial with Ag filling ratiof=0.54. The refractive indices of Ag and SiO2are taken from refs36,37, respectively. (c) EMT-derived dispersion relations for the proposed Ag/SiO2metamaterial atλ=532 nm andλ=633 nm, for TM polarization. The shadowed region represents the optical bandgap of the hyperbolic metamaterial. Figure 1: Hyperbolic metamaterial composed of alternative Ag and SiO 2 thin layers. ( a ) Schematic diagram of the Ag/SiO 2 metamaterial devices. ( b ) EMT-derived effective permittivity ⊥ and || for metamaterial with Ag filling ratio f =0.54. The refractive indices of Ag and SiO 2 are taken from refs 36 , 37 , respectively. ( c ) EMT-derived dispersion relations for the proposed Ag/SiO 2 metamaterial at λ =532 nm and λ =633 nm, for TM polarization. The shadowed region represents the optical bandgap of the hyperbolic metamaterial. Full size image Narrow-band spatial filter based on hyperbolic metamaterial First, we design and implement a planar hyperbolic metamaterial, which blocks transmission of light impinging directly upon its surface at any angle from free-space, but allows internal propagation of grating-coupled modes having spatial frequencies included within a narrow band of values all significantly exceeding the magnitude of the free-space wavevector, k 0 . The resulting metamaterial is composed of alternating thin, flat layers of Ag (30 nm) and SiO 2 (25 nm). The choice of deep-subwavelength thicknesses for each of individual constituent layers, relative to targeted operation wavelengths in the green and red, enables the metamaterial to be approximated as an anisotropic effective medium for modes having an effective wavelength component normal to the layers, which is small compared with the individual layer thicknesses. The electromagnetic response of the metamaterial under this assumption is modelled by an effective magnetic permeability equal to its free-space value, μ eff =1, and a diagonal complex effective-permittivity tensor , where and are the respective complex permittivity components for propagating field components perpendicular and parallel to the axis of anisotropy (here the axis perpendicular to the layers). Using effective medium theory (EMT) [31] , ⊥ and || are calculated ( Fig. 1b ) for the particular case of TM polarization (defined here as the polarization having a magnetic field orientation parallel to the planes of the layers), as and , where Ag and are the dielectric constants of the Ag and SiO 2 , respectively, and f is the filling fraction of Ag. Setting f =0.54, yields opposite signs for and across the visible range. We then analyze the propagation of TM-polarized plane waves at an arbitrary angle within the metamaterial. Choosing a Cartesian coordinate system oriented such that planes of the layers are parallel to the x-y plane, and the wavevector of the incident plane wave lies in the x-z plane, the dispersion relation of the effective medium is given by , where and are the complex amplitudes of the transverse and normal components of the complex wavevector k . Because and , the medium is governed by a hyperbolic equi-frequency curve ( Fig. 1c ) allowing propagation only for modes with wavevectors having , where represents the cutoff transverse spatial frequency. Modes with transverse wavevectors located within the bandgap, , decay evanescently in the z direction. The decay length normal to the layers is given by for modes launched with a uniform phase in the plane of the layers. For free-space wavelengths λ 0 =532 and 633 nm, respective decay lengths l =420 and 385 nm imply that a choice of total metamaterial thickness d =550 nm is sufficient for virtually complete blocking of such a mode. 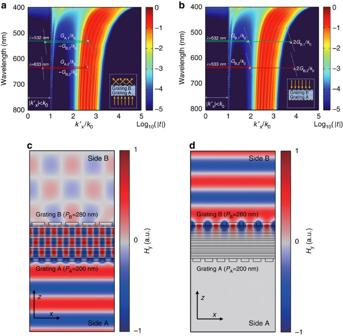Figure 2: Numerical simulations of asymmetric optical transmission with Ag/SiO2metamaterial. (aandb) TMM-calculated magnitude (logarithmic scale) of the electromagnetic field transmission coefficient, |t|, for a free-standing metamaterial stack composed of 10 bilayers of Ag (30 nm) and SiO2(25 nm), for TM-polarized light. Grey dashed lines inarepresent grating vectorsGA−GB(left) andGA(right) for device 1 and devices 2, respectively. Grey dashed lines inbrepresent grating vectorsGB(left) and 2GB(right) for device 1 and device 2, respectively. The corresponding grating pitches arePA,1=200 nm andPB,1=280 nm (device 1),PA,2=240 nm andPB,2=320 nm (device 2). The green and red arrows illustrate the grating-assisted coupling and transmission process of a normally incident plane wave along the direction from (a) side A to side B and (b) side B to side A. (c,d) FDTD-simulated amplitude of they-component of the magnetic field (linear scale) at an arbitrary time, for device 1 illuminated with a TM-polarized plane wave atλ=532 nm for (c) A-to-B and (d) B-to-A. The periodicities of bottom and top gratings are 200 nm and 280 nm, respectively. Figure 2a displays the magnitude of the electromagnetic field transmission coefficient, | t |, of a 550 nm-thick metamaterial stack consisting of 20 alternating layers of Ag (30 nm) and SiO 2 (25 nm), calculated for TM-polarized light illumination in free-space using the transfer matrix method (TMM) [32] , and plotted on a logarithmic colour scale as a function of both the normalized real component of the transverse wavevector, and the free-space wavelength λ 0 in the positive half of the k -space. At all considered values of λ 0 , the function is characterized by a negligible amplitude for , consistent with the hyperbolic transmission bandgap predicted by EMT. As increases above 2 k 0 , increases sharply, consistent with the transition from optical bandgap to hyperbolic transmission band. As increases above 3 k 0 , however, the TMM-calculated value of decreases once again to negligible amplitudes, an effect not predicted under the EMT homogenization approximation. At such high values of , the real normal wavevector component, is also large (consistent with hyperbolic dispersion) and the effective wavelength along the z direction becomes comparable to the individual thicknesses of the Ag and SiO 2 layers. Above this point in k -space, the EMT homogenized metamaterial approximation breaks down, and the material presumably takes on the characteristics of a multilayer scatterer, which is effective at blocking transmission, as a result of its high density of distributed metal reflectors. The basic evolution of the optical transmissivity of the metal-dielectric stack as a function of , including the formation of a transmission band, can be further understood by numerical finite-difference-time-domain (FDTD) simulations of the electromagnetic field profile ( Supplementary Fig. 1 ). Figure 2: Numerical simulations of asymmetric optical transmission with Ag/SiO 2 metamaterial. ( a and b ) TMM-calculated magnitude (logarithmic scale) of the electromagnetic field transmission coefficient, | t |, for a free-standing metamaterial stack composed of 10 bilayers of Ag (30 nm) and SiO 2 (25 nm), for TM-polarized light. Grey dashed lines in a represent grating vectors G A −G B (left) and G A (right) for device 1 and devices 2, respectively. Grey dashed lines in b represent grating vectors G B (left) and 2 G B (right) for device 1 and device 2, respectively. The corresponding grating pitches are P A,1 =200 nm and P B,1 =280 nm (device 1), P A,2 =240 nm and P B,2 =320 nm (device 2). The green and red arrows illustrate the grating-assisted coupling and transmission process of a normally incident plane wave along the direction from ( a ) side A to side B and ( b ) side B to side A. ( c , d ) FDTD-simulated amplitude of the y -component of the magnetic field (linear scale) at an arbitrary time, for device 1 illuminated with a TM-polarized plane wave at λ =532 nm for ( c ) A-to-B and ( d ) B-to-A. The periodicities of bottom and top gratings are 200 nm and 280 nm, respectively. Full size image Figure 2a thus illustrates the formation of a distinct transmission band in k -space, defined here as the range over which | t |>0.1 (where k L and k U represent lower and upper band positions, respectively). For λ 0 ≥500 nm, the band is characterized by a width and center position ( ), which are both relatively constant as a function of free-space wavelength λ 0 . At λ 0 =532 nm and 633 nm, for example, TMM calculations yield lower transmission band-edge values k L ≈2.4 k 0 and k L ≈2.3 k 0 , respectively, which closely match those cutoff frequencies calculated using the EMT approximation ( Fig. 1c ). The corresponding upper transmission band-edge positions calculated by the TMM at those two wavelengths are k U ≈3.1 k 0 and k U ≈3.0 k 0 , respectively. Asymmetric transmission through grating-coupled metamaterial To realize asymmetric optical transmission, we exploit the ability of the metamaterial to block zero-order transmission and transport only waves with large values of the transverse wavevector that furthermore are located within a narrow spatial-frequency band. Though the metamaterial is intrinsically bi-directional and reciprocal along any given direction that sustains propagation, asymmetric transmission of free-space plane waves can be achieved by adding symmetry-breaking metallic gratings to either surface of the metamaterial, which interact with modes inside the metamaterial via evanescent, near-field coupling. Consider a device formed of a block of hyperbolic metamaterial sandwiched by parallel gratings A and B (inset of Fig. 2a,b ), having respective pitches P A and P B and fundamental reciprocal lattice wavevectors of respective magnitude G A =2π/ P A and G B =2π/ P B . G A is chosen to couple normally incident light into a propagating wave in the metal-dielectric stack having a transverse wavevector located just inside the transmission band of the metamaterial . G B is then chosen to make the coupling process at grating B satisfy two simultaneous conditions required by the goal of a asymmetric transmission device. First, to enable coupling of the wave arriving through the metamaterial from side A to an outgoing wave on side B (having tangential wavevector ), G B must satisfy the condition . Second, in order to block transmission into the metamaterial of normally incident light on side B, G B is chosen to avoid coupling to propagating modes of the metamaterial, by forbidding momentum transfer by either fundamental ( ) or higher-order reciprocal grating vectors . Given the k -space position of the single transmission band of the metamaterial, this can be achieved by satisfying the simultaneous constraints G B < k L and 2 G B > k U . Note that the zero-order component of light transmitted by either grating A or B is blocked by the metamaterial. We design two asymmetric transmission devices, one targeted for operation at λ 0 =532 nm (device 1), the other for operation at λ 0 =633 nm (device 2), both incorporating an identical, 550 nm-thick slab of as-designed Ag/SiO 2 hyperbolic metamaterial. Following the coupling principles discussed above, the pitches of gratings A and B are set to, respectively, P A,1 =200 nm and P B,1 =280 nm (device 1) and P A,2 =240 nm and P B,2 =320 nm (device 2). The process of transmission from side A to side B is shown in Fig. 2a for both devices (with green arrows representing in- and out-coupling in the case of device 1 and red arrows representing the equivalent process in the case of device 2). Here for the purposes of illustration, we concentrate on the transmission mechanism though device 1, when side A is illuminated at normal incidence with a plane wave of wavelength λ 0 =532 nm matching the targeted operation wavelength. Grating A couples the incident light into the metamaterial through the action of fundamental grating wavevector G A,1 =2π/ P A,1 =2.66 k 0 (illustrated by the right-directed green arrow) yielding a pair of two, oblique, symmetric, laterally counter-propagating modes having respective tangential real wavevector components which fall within the transmission band of the metamaterial, . These two modes propagate to the other side of the metamaterial, where they are out-coupled into free-space by grating B through the action of fundamental grating wavevector G B,1 =2π/ P B,1 =1.9 k 0 (illustrated by left-directed green arrow), generating a pair of symmetric, laterally counter-propagating plane waves having tangential wavevector k x =±( G A,1 − G B,1 )=±0.76 k 0 , corresponding to propagation angles with respect to the normal of (generating interference fringes of periodicity 350 nm normal to the plane of the device). The process of blocked transmission from side B to side A is shown in Fig. 2b for both devices. For the purposes of illustration, we concentrate on the case of device 1 subject to illumination on side B by a plane wave of wavelength λ 0 =532 nm. Under the assumption of normal incidence, the fundamental grating wavevector G B,1 =1.9 k 0 falls short of lower band edge k L =2.4 k 0 ( G B,1 < k L ) and is thus unable to couple the incident light into the transmission band of the metamaterial. Moreover, the second-order grating wavevector 2 G B,1 (potentially significantly present in the spatial-frequency decomposition of a grating with a Cartesian cross-section) is also unable to couple the incident light to a propagating mode in the metamaterial, since it overshoots the upper edge of the transmission band, k U =3.1 k 0 (2 G B,1 =3.8 k 0 > k U ). Thus, as is clear from Fig. 2b , suppression of normal-incidence in-coupling on side B to a propagating mode in the metamaterial is critically dependent on the formation of a transmission band for that is centred within the interval [ G B,1 , 2 G B,1 ] over a bandwidth smaller than G B,1 . As mentioned earlier, such a band is not achievable with an ideal hyperbolic metamaterial alone (since such a material can sustain propagation for arbitrarily large values of ); the formation of a forbidden band in a range is the direct outcome of the breakdown of the homogeneous medium approximation as the effective wavelength in the metamaterial becomes comparable to the discrete layer thicknesses chosen for the metal/dielectric stack. Indeed, TMM calculations ( Supplementary Fig. 2 ) reveal that the upper transmission band-edge position, k U , is a monotonically decreasing function of Ag/SiO 2 pair layer thickness, d p (at fixed filling ratio of f =0.54 for the Ag, and at fixed total stack thickness of 550 nm), while the lower band edge k L remains constant as a function of t p , at the EMT-predicted value. Setting layer pair thickness to d p =55 nm then yields an upper band edge k U satisfying the blocking condition G B,1 < k U <2 G B,1 . The design approach outlined above for achieving asymmetric transmission via the combination of a hyperbolic metamaterial spatial filter and two gratings with different periods is validated by full electromagnetic simulations using the FDTD method. Figure 2c,d represents the simulated amplitude of the y -component of the magnetic field resulting from illumination of device 1 by a TM-polarized plane wave ( λ 0 =532 nm), normally incident from side A and B, respectively. The constituent individual layer thicknesses (Ag: 30 nm; SiO 2 : 25 nm) and total thickness (550 nm) of the metamaterial are taken to be the same as in the TMM calculations of Fig. 1b,c and Fig. 2a,b . Gratings A and B are taken to be formed in an optically-opaque 50 nm-thick Cr film, with 70 nm-wide rectangular opening, with periods P A,1 =200 nm and P B,1 =280 nm equal to those assumed in Fig. 2a,b . When light is incident on device 1 from side A, it is coupled into the metamaterial by grating A, transmitted through the metamaterial, and then coupled out of the metamaterial by grating B, with significant magnetic field amplitude at each step of the way ( Fig. 2c ), yielding an intensity transmission coefficient into the far field on side B of T A→B ≈−14 dB. Further TMM calculations show that the internal absorption loss of electromagnetic waves ( λ 0 =532 nm) at (corresponding to the magnitude of fundamental grating wavevector G A,1 =2π/ P A,1 =2.66 k 0 ) in the metamaterial over a distance of 550nm normal to the plane of the layers is about −4 dB, implying that the total FDTD-calculated insertion loss corresponding to the present device design is dominated by a combined grating in- and out-coupling efficiency around −10 dB. Magnetic field interference fringes with periodicity of 350 nm are visible on side B, consistent with interference between laterally counter-propagating emerging orders diffracted by grating B. In contrast, when light is incident from side B, a vanishingly small field amplitude is transmitted into the metamaterial owing to inhibited coupling enforced by grating B. As a result, light transmission through device 1 is essentially blocked, with an intensity transmission coefficient into the far field on side B of negligible magnitude T B→A ≈−49 dB. The corresponding contrast ratio for forward versus reverse transmission is then given by γ = T A→B / T B→A ≈35 dB, which confirms highly asymmetric transmission characteristics at normal incidence. FDTD simulations of the device under plane wave illumination at normal incidence show that the transmitted field is independent of lateral position x (that is, along the direction parallel to the plane of the metamaterial layers). Thus, the asymmetric transmission performance of the device is independent of the local lateral phase shift between the two gratings (which varies as a function of x owing to dissimilar grating periods), a combined result of the grating pitch taking on subwavelength values and of the laterally homogeneous nature of the metamaterial stack, which provides translation invariance of its spatial filtering properties (including zero-order transmission blocking). Here the absence of stringent lateral grating-alignment specifications, such as required to date, for example, for THz- or IR-range high-contrast asymmetric transmission schemes based on free-space coupled grating pairs [5] , [11] enables straightforward device fabrication at the sub-micrometre scales required for visible-frequency operation. Moreover, further TMM calculations ( Supplementary Fig. 2 ) show that the metamaterial fully blocks TE-polarized light (having out of plane magnetic field, with respect to the plane of the layers) diffracted into the multilayer stack, for all values of transverse wavevector . In particular, this implies that small angular alignment errors between a given grating orientation and the polarization of light incident on that grating will not significantly affect the forward-to-reverse transmission contrast ratio. This stands in contrast to grating-polarizer-based asymmetric transmission device [6] , for which a high transmission contrast ratio is critically dependent on the polarization angle of the incident light with respect to the grating orientation. Experimental demonstration at visible frequencies The grating-coupled metamaterial designs optimized above for asymmetric operation in air at λ 0 =532 nm (device 1) and at λ 0 =633 nm (device 2) are fabricated in the form of two free-standing devices using a silicon-nitride membrane as a starting substrate (see Methods for details of the fabrication process). A combination of sputter deposition and focused-ion-beam (FIB) milling is used to form a 550 nm-thick Ag/SiO 2 , multilayer metamaterial core (consisting of alternating layers of Ag and SiO 2 with targeted thickness of 30 nm and 25 nm, respectively), bearing back-to-back 10 μm × 10 μm patches of parallel, air-facing periodic surface gratings patterned into 50 nm-thick Cr films located on either side of the metamaterial, as shown in Fig. 3a (denoted side ‘A’ and ‘B’, respectively, where A→B is the designed direction of high transmissivity under normal-incidence illumination). Fixed grating aperture width (≈70 nm) and variable periods of the fabricated gratings are chosen to match those of the two optimized designs (namely, P A,1 =200 nm and P B,1 =280 nm in the case of device 1, and P A,2 =240 nm and P B,2 =320 nm in the case of device 2). To characterize their optical performance, devices 1 and 2 are illuminated with TM-polarized, bandpass-filtered super-continuum laser light (10 nm full-width at half-maximum), at centre wavelengths of λ 0 =532 nm (device 1) and λ 0 =633 nm (device 2), respectively. The transmitted light is collected and imaged using an inverted optical microscope with a × 100 objective lens (numerical aperture=0.9) and a Si charge-coupled device (CCD) camera. The narrow-band spectral dependence of the as-collected forward and reverse transmitted intensities, I A→B ( λ ) and I B→A ( λ ), normalized to transmitted intensity at λ 0 , I A→B ( λ 0 ), are displayed in Fig. 3b,c for each device, along with the corresponding optical images of the respective device exit surfaces. Measured transmission contrast ratios γ ( λ 0 )≡ I A→B ( λ 0 )/ I B→A ( λ 0 ) of 15.3 dB for device 1 at λ 0 =532 nm, and 14.4 dB for device 2 at λ 0 =633 nm confirm high-contrast asymmetric optical transmission. These values are somewhat lower than those predicted by FDTD simulations (respectively 35 and 34 dB), possibly owing to dimensional or morphological deviations in the structure of the fabricated devices compared with that of the ideal model structures (such as deviations in the thickness or flatness of the individual layers of the metamaterial stack, which are affected by the grain structure of the deposited Ag). The exit-side images of Fig. 3b exhibit interference fringes with respective periodicities of ≈350 nm (device 1) and ≈480 nm (device 2) that agree well with theoretical calculations and FDTD simulations, confirming that transmitted light emerges into the far field under the form of laterally counter-propagating orders at angles of 49.5° (device 1) and 41.3° (device 2). 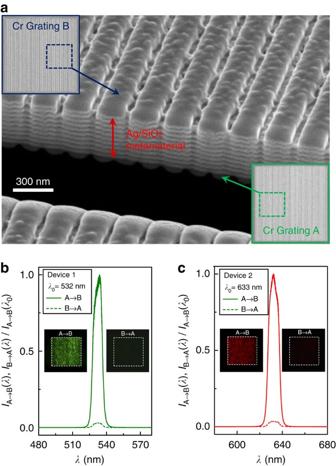Figure 3: Experimental demonstration of asymmetric optical transmission through grating-coupled metamaterial devices. (a) Scanning electron microscope (SEM) image of fabricated experimental device 1, cross-sectioned by FIB milling to reveal the internal metamaterial structure. Left inset, SEM image of top Cr grating with 280 nm periodicity (lateral dimensions: 10 μm × 10 μm). Right inset, SEM image of bottom Cr grating with 200 nm periodicity (lateral dimensions identical to those of top grating). (bandc) Measured forward and backward transmitted intensities for device 1 (b) and device 2 (c) atλ=532 nm and 633 nm, respectively. The incident illumination consists of normally incident TM-polarized super-continuum light that is bandpass filtered (bandwidth: 10 nm) at centre wavelengths of 532 nm (device 1) and 633 nm (device 2). Insets, optical-microscope image of exit sides of devices 1 and 2, under forward and reverse transmission at designed wavelengths of operation. Figure 3: Experimental demonstration of asymmetric optical transmission through grating-coupled metamaterial devices. ( a ) Scanning electron microscope (SEM) image of fabricated experimental device 1, cross-sectioned by FIB milling to reveal the internal metamaterial structure. Left inset, SEM image of top Cr grating with 280 nm periodicity (lateral dimensions: 10 μm × 10 μm). Right inset, SEM image of bottom Cr grating with 200 nm periodicity (lateral dimensions identical to those of top grating). ( b and c ) Measured forward and backward transmitted intensities for device 1 ( b ) and device 2 ( c ) at λ =532 nm and 633 nm, respectively. The incident illumination consists of normally incident TM-polarized super-continuum light that is bandpass filtered (bandwidth: 10 nm) at centre wavelengths of 532 nm (device 1) and 633 nm (device 2). Insets, optical-microscope image of exit sides of devices 1 and 2, under forward and reverse transmission at designed wavelengths of operation. Full size image Slabs of hyperbolic metamaterial decorated with diffraction gratings enable high-contrast asymmetric transmission not only at a specific wavelength, but also across a relatively broad spectral range. For example, Fig. 4 plots the forward and reverse intensity transmission coefficients, respectively T A→B and T B→A measured for both devices 1 and 2 as a function of free-space wavelength λ . The respective wavelength spans corresponding to a transmission contrast ratio γ ≥10 dB are 83 nm for device 1 (covering wavelength range 508–590 nm), and 117 nm for device 2 (covering wavelength range 572–688 nm). This implies for each device a fractional bandwidth >15% for asymmetric transmission contrast >10:1. This relatively large wavelength bandwidth for grating in- and out-coupling with a propagating metamaterial mode is enabled by a spatial-frequency passband of the constituent metamaterial, which is both relatively wide as a function of k x and relatively vertical as a function of λ ( Fig. 2a,b ). 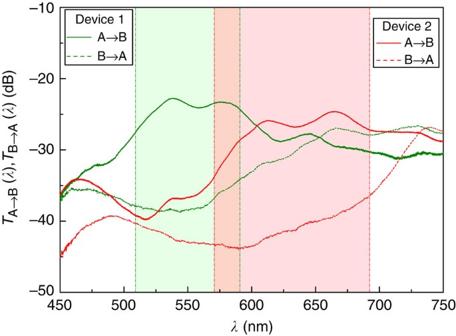Figure 4: Broadband asymmetric response of the fabricated devices. Measured A-to-B and B-to-A intensity transmission coefficients for device 1 and device 2, respectively, across the visible spectrum. The green and red shadows indicate the respective device regions over which the forward/reverse transmission contrast ratio,γ, is higher than 10 dB. Figure 4: Broadband asymmetric response of the fabricated devices. Measured A-to-B and B-to-A intensity transmission coefficients for device 1 and device 2, respectively, across the visible spectrum. The green and red shadows indicate the respective device regions over which the forward/reverse transmission contrast ratio, γ , is higher than 10 dB. Full size image For A to B transmission, the insertion losses (device intensity transmission coefficients) for device 1 and device 2 at designed operation wavelengths of λ 0 =532 nm and λ 0 =633 nm are −23 dB and −26.5 dB, respectively. These high insertion losses are assumed to result from both internal absorption in the constituent layers of the metamaterial, as well as sub-optimal in- and out- grating coupling. We expect that the grating coupling efficiencies can be significantly improved by tuning the grating shape to maximize the fundamental grating wavevector with respect to the higher-order grating wavevector components. Absorption losses, on the other hand, may potentially be compensated by imbedding an active gain in within the dielectric layers of the metamaterial [33] , [34] , [35] . Although we experimentally demonstrate asymmetric optical transmission for normally incident plane waves, the grating-coupled metamaterial devices are also theoretically able to enforce asymmetric transmission over a wide range of incident angles about the normal, owing to the finite lateral spatial-frequency transmission bandwidth of the hyperbolic metamaterial, of width≈ k 0 . Given an incident angle θ , asymmetric optical transmission from side A to side B simultaneously requires the respective in- and out-coupling conditions given by k L <| G A + k 0 sin θ |< k U , | G B + k 0 sin θ |< k L and | 2 G B + k 0 sin θ |> k U . Solution of this system yield angular ranges of incidence satisfying asymmetric transmission of ±15° and ±19° relative to the normal, for device 1 and 2, respectively. In conclusion, we have designed and experimentally demonstrated a passive, time-independent metamaterial-based device able to enforce highly asymmetric transmission of visible light. Broadband asymmetric transmission is realized by combining a hyperbolic metamaterial able to act as a pass-band filter for high spatial frequencies beyond the diffraction limit, with a pair of nonsymmetric, subwavelength-period gratings able to couple into and out of a propagating mode in the material, upon normal-incidence illumination of only one of the two gratings. Thanks to its planar architecture and low-footprint, this asymmetric transmission metamaterial device appears promising for use in integrated optical systems operating at visible frequencies. To fabricate the free-standing grating-decorated metamaterial devices, bottom Cr, Ag/SiO 2 metamaterial and top Cr layers were subsequently deposited on a silicon-nitride (Si 3 N 4 ) membrane by physical sputtering in the same sputter chamber. The sputter-deposition rates for Cr, Ag and SiO 2 were R Cr ≈3 Å s −1 , R Ag ≈3.6 Å s −1 and , respectively. FIB milling (Ga+ ions, 30 keV) was then used from the membrane side to locally remove the Si 3 N 4 and pattern a 10 μm × 10 μm grating structure into the bottom Cr layer. Reference alignment marks through the full thickness of the metamaterial and Cr layers were also patterned by FIB milling in the vicinity of the bottom grating structure. Finally, the sample was flipped over and another 10 μm × 10 μm grating was patterned by FIB milling into the top Cr layer, with the same grating orientation and at the same lateral position as the bottom grating, as inferred from the alignment marks. How to cite this article: Xu, T. and Lezec, H. J. Visible-frequency asymmetric transmission devices incorporating a hyperbolic metamaterial. Nat. Commun. 5:4141 doi: 10.1038/ncomms5141 (2014).